Nucleophilic arylation with tetraarylphosphonium salts Organic phosphonium salts have served as important intermediates in synthetic chemistry. But the use of a substituent on the positive phosphorus as a nucleophile to construct C–C bond remains a significant challenge. Here we report an efficient transition-metal-free protocol for the direct nucleophilic arylation of carbonyls and imines with tetraarylphosphonium salts in the presence of caesium carbonate. The aryl nucleophile generated from phosphonium salt shows low basicity and good nucleophilicity, as evidenced by the successful conversion of enolizable aldehydes and ketones. The reaction is not particularly sensitive to water, shows wide substrate scope, and is compatible with a variety of functional groups including cyano and ester groups. Compared with the arylmetallic reagents that are usually moisture sensitive, the phosphonium salts are shelf-stable and can be easily handled. Significant advances in C-arylation have emerged in the past few decades because this reaction can effectively form C–C bonds to provide valuable molecules that are the core structures of natural products or pharmaceuticals [1] , [2] , [3] , [4] , [5] . Recently, intensive studies have been devoted to the exploration of efficient methods for arylation of carbonyl and imino compounds, allowing access to α-aryl-alcohols and α-aryl-amines, which are abundant in biologically active molecules [1] , [2] . Traditional arylmetallic reagents, which are usually generated in situ under Barbier-type conditions [6] , [7] , [8] or prepared in advance like arylmagnesium reagents [9] , [10] , [11] , have long been used for nucleophilic addition to carbonyl or imino groups. However, this approach often suffers from narrow substrate scope, or the high moisture sensitivity and the strong basicity of the reagents. Transition-metal-catalysed arylation of carbonyl or imino groups with aryl halides [12] , [13] , arylboronic acid derivatives [14] , [15] , [16] , [17] , [18] , [19] , [20] or other reactive reagents [21] , [22] , [23] , [24] , [25] showed good functional group tolerance under mild reaction conditions. However, the high cost of noble transition metal complexes and possible contamination of the end products by trace amounts of heavy metals probably limit the wide application of this approach in industrial and pharmaceutical processes. Therefore, it is highly desirable to explore broadly applicable transition-metal-free methods for the arylation of carbonyl and imino compounds. Our research interest in the chemistry of organic phosphonium salts [26] , [27] , [28] , [29] prompted us to investigate their application in arylation reactions. Organic phosphonium salts have served as important intermediates in synthetic chemistry [30] , [31] , [32] , [33] , [34] , [35] . Although phosphonium salts are electrophilic species and the positive phosphorus could enhance the electrophilicity [36] or acidity [34] , [35] , [37] of its substituents because of the inductive effect, we speculated that the substituent on the phosphorus might be converted to a nucleophile initiated by another appropriate nucleophile, which may firstly attack the phosphorus and then result in the cleavage of a substituent with nucleophilic ability ( Fig. 1 ). 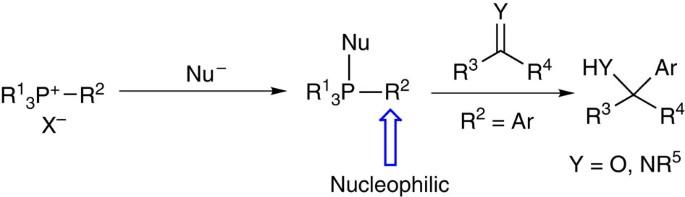Figure 1: Design of arylation reaction with phosphonium salt. An aryl substituent on phosphorus can act as a nucleophile to realize the nucleophilic arylation of carbonyls and imines. Figure 1: Design of arylation reaction with phosphonium salt. An aryl substituent on phosphorus can act as a nucleophile to realize the nucleophilic arylation of carbonyls and imines. Full size image Herein we report a nucleophilic arylation of carbonyl and imino compounds with tetraarylphosphonium salts in the presence of caesium carbonate ( Fig. 1 ). The generated aryl nucleophiles exhibit low basicity and good nucleophilicity. The arylation protocol shows wide substrate scope and a high level of functional group tolerance. Mechanistic investigation reveals that the reaction is predominantly initiated by caesium carbonate. Optimization of reaction conditions Considering the high affinity between phosphorus and oxygen, an O-nucleophile was used to initiate the arylation of 4-phenylbenzaldehyde ( 1a ) with tetraphenylphosphonium iodide ( 2a ) ( Table 1 , entries 1–4). Neither Na 2 CO 3 nor K 2 CO 3 could initiate the transformation (entries 1 and 2). Interestingly, Cs 2 CO 3 was found to be a good initiator (entry 3), which is likely because of the better solubility of the caesium salt. Because the caesium salt was effective, another O-initiator with caesium as the cation (CsOAc; entry 4) was examined. To our surprise, no desired product was detected, which might be caused by the lower nucleophilicity of the acetate anion. Further screening of non-O-initiators (entries 5 and 6) showed that Cs 2 CO 3 was the best initiator (entry 3), indicating that the high P–O affinity may have an important role in this reaction. The yield was increased to 65% with the elongation of reaction time (entry 7 versus entry 3). The effects of other solvents were also investigated (entries 8–10). The reaction in 1,4-dioxane gave the product in comparable yield (entry 8 versus entry 7), while acetonitrile was not as effective, probably because its acidic α-proton can quench the leaving phenyl group from salt 2a (entry 10). Increasing the loading of salt 2a and caesium carbonate (entries 11 and 12) increased the yield significantly (entry 12), while lowering the temperature led to significantly lower yield (entry 13). The reaction was not particularly sensitive to water, as evidenced by the moderate yield obtained with the addition of water into the reaction system (entry 14). Both of the chloride (Ph 4 P + Cl − ) and bromide (Ph 4 P + Br − ) instead of the iodide 2a gave lower yields, which should be due to the lower solubility of the chloride and bromide (entries 15–16). Table 1 Screening reaction conditions * . 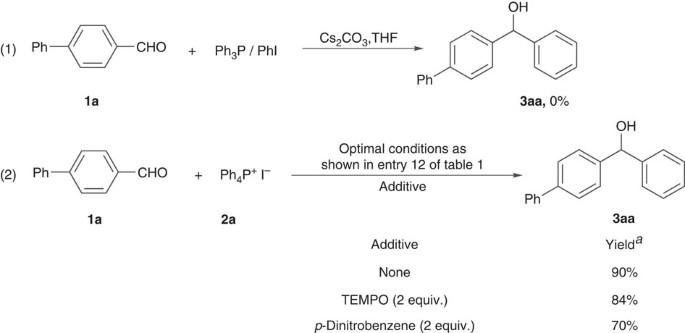Figure 2: Mechanistic experiments. (1) The use of Ph3P/PhI system instead of salt2afailed to convert aldehyde1ainto product3aa. (2) Neither radical scavenger TEMPO nor single-electron-transfer inhibitorp-dinitrobenzene can obviously suppress the phenylation reaction.aIsolated yields. Full size table Substrate scope for phenylation of aldehydes With the optimized reaction conditions in hand ( Table 1 , entry 12), we then explored the substrate scope for the phenylation of aldehydes with phosphonium salt 2a ( Table 2 ). The transformation can be applied to a variety of aldehydes and gave the desired products in moderate to excellent yields. Increasing the scale of the reaction by 20-fold still afforded the desired product 3aa in good yields, which is highly important in the synthetic application, albeit the longer reaction time or higher loading of Cs 2 CO 3 was required. Investigation of the electronic effects showed that the electron-donating or -withdrawing groups on the aryl ring did not significantly influence the reaction ( 3aa – 3ra ). A broad functionality tolerance was demonstrated for aryl aldehydes bearing different substituents, including cyano ( 3la – 3ma ) and ester groups ( 3na ). The conversion was not quite sensitive to steric effects, given that high yields were obtained for products 3ea , 3ka and 3oa . It is noteworthy that the enolizable aldehydes were also converted into the expected products in good yields ( 3ta and 3ua ) without self-aldol condensation. Table 2 Substrate scope of phenylation of aldehydes * . 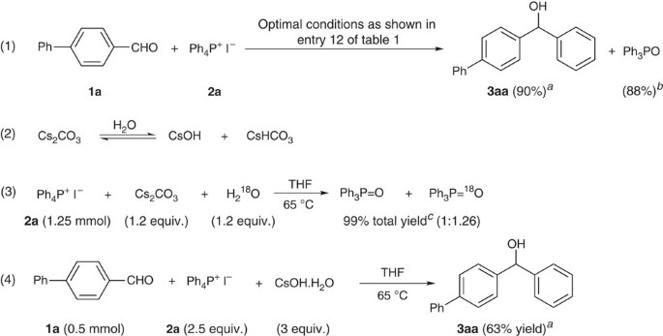Figure 3: Evidence to support the path via alkaline hydrolysis. (1) Ph3PO was isolated as a by-product for phenylation reaction.aIsolated yield based on1a;bIsolated yield based on2a; (2) An equilibrium between Cs2CO3and CsOH may be established under the reaction conditions. (3) The presence of H218O led to the formation of Ph3P18O.cIsolated yield. (4) CsOH can also initiate the phenylation reaction. Full size table Substrate scope for phenylation of ketones Although ketone is less reactive than aldehyde, the phenylation of ketones with salt 2a still proceeded smoothly to give the desired products ( Table 3 ). However, increased loading of salt 2a and caesium carbonate to 4 and 4.5 equivalents, respectively, was necessary to achieve good yields. Both aromatic ( 5a – 5l ) and aliphatic ketones ( 5m and 5n ) were reactive under the optimal conditions. The successful conversion of hindered ketones indicates that the reaction is moderately tolerant to steric effects ( 5f – 5h , 5j ). In addition, no reaction at the carbonyl-activated ester group of 5k suggests that the transformation shows high chemoselectivity. Table 3 Substrate scope of phenylation of ketones * . Full size table Compared with the traditional arylation of carbonyl groups with arylmetallic reagents, which are strong nucleophiles and can lead to the arylation of cyano [38] and ester [12] groups, this mild reaction clearly exhibits a higher level of functional group tolerance. More importantly, the reaction is applicable to enolizable aldehydes and ketones, indicating that the in situ -generated phenyl-anion equivalent exhibits high nucleophilicity and low basicity. 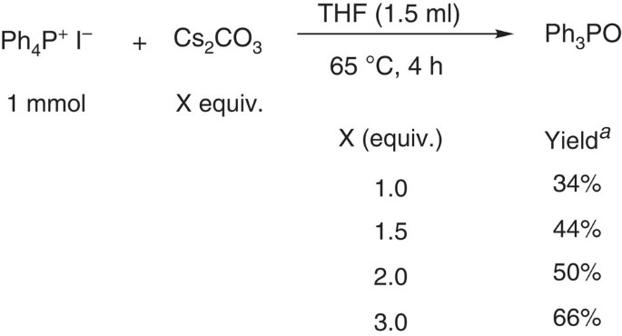Figure 4: Evidence to support the Cs2CO3promoted arylation without water. The more Cs2CO3was used for the reaction of Ph4P+I−with Cs2CO3for the same period of time, the more Ph3PO was produced,ayields were determined by31P NMR. Substrate scope for phenylation of imines The successful conversion of aldehydes and ketones prompted us to examine the phenylation of imines with salt 2a ( Table 4 ). Imines containing electron-donating groups on the phenyl ring were effectively converted into the desired products, but for imines with a strong electron-withdrawing substituent such as cyano, the reaction failed to give the desired product. It is likely that under these reaction conditions, the imine is prone to hydrolysis to give the aldehyde, which would then react with salt 2a to afford the alcohol. In contrast to tosyl-protected imines ( N -Ts), p -methoxyphenyl-protected imine ( N -PMP) is inert under the reaction conditions. Table 4 Substrate scope of phenylation of imines * . Full size table The investigation of the reactivity of phosphonium salts The reactivities of different tetraarylphosphonium salts were also investigated. 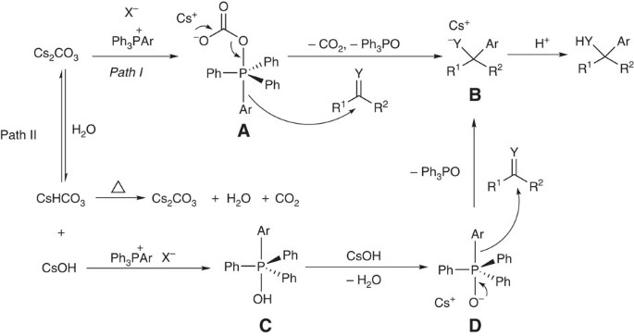Figure 5: Proposed nucleophilic arylation mechanism. The reaction should be predominantly initiated by Cs2CO3(path I), and may also be promoted by CsOH due to the trace amount of water present in the reaction system (path II). Compared with tetraphenylphosphonium iodide ( 3aa , Table 2 ), tetra- p -methoxyphenylphosphonium iodide ( Table 5 , entry 1) and tetra- p -methylphenylphosphonium iodide (entry 2) showed lower reactivity towards arylation and gave the corresponding arylation products in lower yields. This is probably because the in situ -generated aryl-anion equivalent containing an electron-donating group is less stable and would readily abstract a proton from the trace amount of water present. Table 5 Substrate scope of arylation of 4-phenylbenzaldehyde * >. Full size table To this point of our study, the four aryl groups on the phosphorus were identical. It will be interested to know the different leaving ability when one aryl group was different from the others. To address this issue, a variety of aryl triphenylphosphonium salts were prepared and tested for the arylation of aldehyde 1a ( Table 5 , entries 3–9). If the aryl moiety contained a weak electron-withdrawing group, the corresponding arylation product was obtained in low yield (entry 3), with simultaneous formation of more phenylation product 3aa (43% yield). This might be because the leaving ability between the phenyl and aryl group is similar owing to their comparable electron-withdrawing effect, and three phenyl groups compete with one aryl group, thus leading to more phenylation product 3aa . However, if the aryl moiety was substituted with a strong electron-withdrawing group, the phenylation product 3aa would be greatly suppressed and the arylation became the main reaction, indicating that electron-withdrawing ability has an important role in the selectivity (entries 4–7). In the case of 3ai , the low yield was not because of the phenylation reaction to produce 3aa , but because of a side reaction to give 4′-phenylacetophenone (27% yield based on aldehyde; entry 8). Pyridyl triphenylphosphonium iodide was also suitable for the desired pyridylation (entry 9). In the case of the salts containing strong electron-withdrawing groups ( 2e′ – 2i′ ), it would be better to change the salt anion from iodide to bis(trifluoromethanesulfonyl)imide anion (Tf 2 N − ) and the procedure for arylation should be modified accordingly. For example, the in situ -generated aryl-anion equivalent would readily attack the phosphonium salt to give the diaryl by-product (33% based on aldehyde) because of the increased electrophilicity of the salt. To avoid this problem, the phosphonium salts were added slowly to the reaction to keep the substrate aldehyde in constant excess. And this required the salts to be soluble in tetrahydrofuran (THF) so as to realize the addition of the salts via syringe. The phosphonium salts containing Tf 2 N − were soluble in THF and the corresponding arylation proceeded smoothly by the addition of the phosphonium salt solution into the reaction ( Table 5 , entries 4–8). Mechanistic investigation As for the reaction mechanism, the analysis of trace transition metal in phosphonium salts and caesium carbonate by ICP spectrometry ( Supplementary Table 1 ) revealed that this arylation is a transition-metal-free reaction. Although salt 2a is quite stable, an equilibrium might be established between this salt and Ph 3 P/PhI under the phenylation conditions. But the use of Ph 3 P/PhI system instead of salt 2a for the phenylation of aldehyde 1a failed to give the desired product at all (equation 1 Fig. 2 ), meaning that the equilibrium cannot account for the arylation. Neither radical scavenger TEMPO [(2,2,6,6-tetramethylpiperidin-1-yl)oxyl] nor single-electron-transfer inhibitor p -dinitrobenzene can dramatically suppress the phenylation of aldehyde 1a with salt 2a , indicating that the arylation may not proceed via a single-electron-transfer mechanism (equation 2, Fig. 2 ). Nothing happened while refluxing aldehyde 1a /salt 2a system or aldehyde 1a /Cs 2 CO 3 system in THF. But the full conversion of salt 2a into Ph 3 PO was observed by refluxing salt 2a and Cs 2 CO 3 in THF, suggesting that the interaction between salt 2a and Cs 2 CO 3 initiates this arylation reaction. Figure 2: Mechanistic experiments. (1) The use of Ph 3 P/PhI system instead of salt 2a failed to convert aldehyde 1a into product 3aa . (2) Neither radical scavenger TEMPO nor single-electron-transfer inhibitor p -dinitrobenzene can obviously suppress the phenylation reaction. a Isolated yields. Full size image The alkaline hydrolysis of phosphonium salts has been well-studied for the past decades [30] , [39] , [40] , [41] , [42] , [43] , [44] , [45] , [46] , [47] . As a third-order reaction (first order with respect to phosphonium salt, second order to hydroxide) [40] , [41] , the alkaline hydrolysis of tetraphenylphosphonium salt would lead to the formation of triphenylphosphine oxide (Ph 3 PO) (refs 46 , 48 ). Since Ph 3 PO was detected by gas chromatography mass spectrometry (GC–MS) in every phenylation reaction system using 2a (Ph 4 P + I − ) and Ph 3 PO was isolated in high yield for the phenylation of substrate 1a (equation 1, Fig. 3 ), it is reasonable to conceive that the arylation might proceed via this hydrolysis process. Although the solvent THF purchased from commercial source was extra dry (‘Extra Dry over Molecular Sieve’,<0.005% water content) and the arylation was performed under N 2 atmosphere, trace amount of water may still be unavoidable in the reaction system, thus leading to the hydrolysis of caesium carbonate (equation 2). The resulting hydroxide anion would decompose the phosphonium salt to generate Ph 3 PO, suggesting that the oxygen in Ph 3 PO could partially come from water. Indeed, the reaction of phosphonium salt with caesium carbonate in the presence of H 2 18 O gave both Ph 3 PO and Ph 3 P 18 O (equation 3). The molar ratio of Ph 3 PO: Ph 3 P 18 O determined by 31 P NMR was 1:1.26. This ratio was consistent with elemental analysis of the mixture (see Supplementary Methods for the formation of Ph 3 P 18 O). It seems that this hydrolysis process might be involved in the arylation, which was further supported by the observation that the direct use of caesium hydroxide instead of caesium carbonate also gave the expected product in 63% yield (equation 4). Compared with the 90% yield while using Cs 2 CO 3 , lower yield might result from the presence of hydrated water in CsOH (note: anhydrous CsOH is not commercially available). Although water can promote the hydrolysis of Cs 2 CO 3 to produce CsOH, excessive water would suppress the subsequent arylation through the capture of the in situ -generated phenyl nucleophile. In addition, this possible hydrolysis process of Cs 2 CO 3 could also explain why moderate yield (49%) of phenylation product could be obtained with the deliberate addition of water (entry 14 of Table 1 ). Figure 3: Evidence to support the path via alkaline hydrolysis. (1) Ph 3 PO was isolated as a by-product for phenylation reaction. a Isolated yield based on 1a ; b Isolated yield based on 2a ; (2) An equilibrium between Cs 2 CO 3 and CsOH may be established under the reaction conditions. (3) The presence of H 2 18 O led to the formation of Ph 3 P 18 O. c Isolated yield. (4) CsOH can also initiate the phenylation reaction. Full size image Nevertheless, all reagents including highly dry Cs 2 CO 3 (99.994% purity, metals basis) and the solvent THF (<0.005% water content) were stored in a glove box, and the arylation were conducted under N 2 atmosphere, suggesting that the water content in the reaction system should be extremely low. This trace amount of water cannot cause the complete hydrolysis of Cs 2 CO 3 , indicating that another reaction process should exist. As shown in Table 2 , for the large-scale phenylation to give 3aa , significantly less reaction time (12 h versus 120 h) was needed to achieve comparable yield (75% versus 84%) with the use of more Cs 2 CO 3 (5 equivalents versus 3 equivalents). The water contents (trace) in both reaction systems should be the same since these reactions were conducted under the same reaction conditions. The faster arylation with the use of more Cs 2 CO 3 means that Cs 2 CO 3 may be able to promote the arylation without the involvement of water. If this is the case, more Cs 2 CO 3 would result in a faster conversion of Ph 4 P + I − into Ph 3 PO. Indeed, for the reaction of Ph 4 P + I − with Cs 2 CO 3 in THF for 4 h, the more Cs 2 CO 3 was used, the more Ph 3 PO was produced (note: Ph 4 P + I − was not completely consumed in every reaction; Fig. 4 ). These results indicate that Cs 2 CO 3 , for the most part, directly promoted this arylation. Figure 4: Evidence to support the Cs 2 CO 3 promoted arylation without water. The more Cs 2 CO 3 was used for the reaction of Ph 4 P + I − with Cs 2 CO 3 for the same period of time, the more Ph 3 PO was produced, a yields were determined by 31 P NMR. Full size image Apparently, nucleophilic phenyl species was formed in the process of the arylation. Salt 2a , also as an electrophilic species, might be able to trap this nucleophilic phenyl group to give Ph 5 P (ref. 49 ). To ascertain whether Ph 5 P is generated or not, more evidences were collected. 31 P NMR measurement of the reaction of 1a with salt 2a only detected the formation of Ph 3 PO. Furthermore, instead of the phosphonium salt 2a , Ph 5 P was directly used in its reaction with aldehyde (See Supplementary Methods for the procedure for arylation of 1a with Ph 5 P) [50] , [51] . However, no desired product 3aa was detected without the presence of Cs 2 CO 3 . And even in the presence of Cs 2 CO 3 , the yield of 3aa was very low (11%), indicating that Ph 5 P may not be involved in the above arylation. On the basis of the above results, we proposed a plausible mechanism shown in Fig. 5 . The direct attack of Cs 2 CO 3 at the phosphonium cation is the predominant path (Path I). Nucleophilic addition to the positive phosphorus would always be along the axial co-ordinate and pseudorotation would occur afterwards to place the electronegative substituent in the other axial position [30] , [39] , [47] , [52] , generating trigonal bipyramidal tetraaryloxyphosphorane A . The simultaneous decarboxylation and nucleophilic attack of Ar in intermediates A to carbonyl or imino groups afford Ph 3 PO and the adduct B , which is then protonated by acid to furnish the final product. However, owing to the unavoidable presence of trace amount of water, an equilibrium between Cs 2 CO 3 and CsHCO 3 /CsOH may be established (path II). CsHCO 3 might gradually decompose into Cs 2 CO 3 , water and carbon dioxide at the reaction temperature. The generated CsOH would promote the subsequent arylation via an alkaline-hydrolysis path [30] , [39] , [40] , [41] , [42] , [43] , [44] , [45] , [46] , [47] . Nucleophilic addition of hydroxide to phosphorus and the subsequent pseudorotation generate intermediate C , deprotonation of which by CsOH gives an oxyanionic phosphorane D . The expulsion of the aryl anion from intermediate D and the nucleophilic addition of this Ar group to substrate also afford the adduct B and Ph 3 PO. Therefore, the two paths might coexist. It should be noted that none of the intermediate A , C or D was detected by 31 P NMR, although P -hydroxytetraorganophosphorane has recently been observed and characterized by low-temperature NMR [53] . Considering that cyano and ester groups are stable under the optimized reaction conditions and the enolizable carbonyl compounds were successfully converted, the naked aryl anion is not believed to be formed in the arylation process. Carbon dioxide cannot be detected by GC–MS in the gas phase of the reaction system because the gas phase was full of the solvent THF. Fortunately, when DMF was used instead of THF in the reaction of aldehyde 1a with salt 2a , GC–MS analysis of the gas phase of the reaction mixture successfully detected the generation of CO 2 (see ‘determination of CO 2 by GC–MS spectroscopy’ in Supplementary Methods ) albeit that the desired product was isolated in only 60% yield, further supporting the proposed reaction mechanism. Figure 5: Proposed nucleophilic arylation mechanism. The reaction should be predominantly initiated by Cs 2 CO 3 (path I), and may also be promoted by CsOH due to the trace amount of water present in the reaction system (path II). Full size image Although phosphonium salts are electrophilic species, we found that a substituent on the positive phosphorus can act as a nucleophile for the construction of C–C bond while initiated by another appropriate nucleophile. The successful application of tetraarylphosphonium salts to the nucleophilic transition-metal-free arylation of carbonyl and imino compounds in the presence of caesium carbonate is described herein. The high P–O affinity has an important role in this arylation strategy. This practical protocol is attractive because the reaction is not particularly sensitive to water, shows wide substrate scope under mild conditions, and is compatible with a variety of functional groups. It provides a highly valuable method for C-arylation and easy access to α-aryl-alcohols and α-aryl-amines. In addition, the success of the strategy means that phosphonium salts may find applications in other areas of chemistry. General procedure for phenylation of aldehydes Under N 2 atmosphere, the mixture of aldehyde (0.50 mmol), tetraphenylphosphonium iodide (583.0 mg, 1.25 mmol) and Cs 2 CO 3 (488.7 mg, 1.50 mmol) in THF (4 ml) and stirred at 65 °C for 12 h. The reaction was quenched by 3 N HCl (0.5 ml). The resulting mixture was extracted with dichloromethane (DCM; 3 × 30 ml). The combined organic phase was dried over Na 2 SO 4 . After filtration, the solvent was removed by concentration, and the residue was subjected to column chromatography to afford the pure product. General procedure for phenylation of ketones Under N 2 atmosphere, the mixture of ketone (0.40 mmol), tetraphenylphosphonium iodide (745.8 mg, 1.60 mmol) and Cs 2 CO 3 (586.4 mg, 1.80 mmol) in THF (4 ml) was stirred at 65 °C for 24 h. The reaction was quenched by 4.5 N HCl (1.5 ml). The resulting mixture was extracted with DCM (3 × 30 ml). The combined organic phase was dried over Na 2 SO 4 . After filtration, the solvent was removed by concentration, and the residue was subjected to column chromatography to afford the pure product. General procedure for phenylation of imines Under N 2 atmosphere, the mixture of imine (0.50 mmol), tetraphenylphosphonium iodide (583.0 mg, 1.25 mmol) and Cs 2 CO 3 (488.7 mg, 1.50 mmol) in THF (4 ml) was stirred at 65 °C for 12 h. The reaction was quenched by 3 N HCl (0.5 ml). The resulting mixture was extracted with DCM (3 × 30 ml). The combined organic phase was dried over Na 2 SO 4 . After filtration, the solvent was removed by concentration. The residue was subjected to column chromatography to afford the pure product. Arylation of 1a with various teraarylphosphonium salts Method A. Under N 2 atmosphere, the mixture of [1,1′-biphenyl]-4-carbaldehyde ( 1a ; 91.2 mg, 0.50 mmol), tetraarylphosphonium iodide (1.25 mmol) and Cs 2 CO 3 (488.7 mg, 1.50 mmol) in THF (4 ml) was stirred at 65 °C until phosphonium salt was completely consumed as monitored by 31 P NMR. The reaction was quenched by 3 N HCl (0.5 ml). The resulting mixture was extracted with DCM (3 × 30 ml). The combined organic phase was dried over Na 2 SO 4 , and the residue was subjected to column chromatography to afford the pure product. Method B . Under N 2 atmosphere, into the mixture of [1,1′-biphenyl]-4-carbaldehyde ( 1a ; 91.2 mg, 0.50 mmol) and Cs 2 CO 3 (488.7 mg, 1.50 mmol) in THF (2 ml) at 65 °C was added the solution of phosphonium bis(trifluoromethanesulfonyl)amide (1.25 mmol) in THF (2 ml) slowly for 6 h. On completion of addition, the reaction was stirred for another 10 min. The mixture was quenched by 3 N HCl (0.5 ml) and extracted with DCM (3 × 30 ml). The combined organic phase was dried over Na 2 SO 4 . After filtration, the solvent was removed by concentration, and the residue was subjected to column chromatography to afford the pure product. How to cite this article: Deng, Z. et al . Nucleophilic arylation with tetraarylphosphonium salts. Nat. Commun. 7:10337 doi: 10.1038/ncomms10337 (2016).